‘Fetal side’ of the placenta: anatomical mis-annotation of carbon particle ‘transfer’ across the human placenta 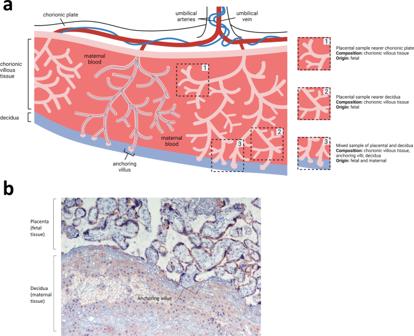Fig. 1: Structure of the term placenta, and biopsy sampling. aThe umbilical vein and arteries containing fetal blood reach the placenta at the cord insertion site and spread across the chorionic plate, branching extensively to provide the tree-like shape of the placenta. The branched vessels are embedded in a stromal core covered by trophoblast cells which are completely bathed in maternal blood within the intervillous space. Anchoring villi attach the placenta to the maternal endometrium (decidua). The three dashed-line boxes indicate the potential biopsy locations utilised by Bove et al. (1) and (2) are standard placental biopsies, comprising chorionic villous tissue that is fetal in origin, whilst excluding contamination with maternal decidual tissue. Regardless of whether a placental biopsy is taken near to the chorionic plate (1) or close to the decidua (2), the tissue is totally fetal. (3) represents an alternative possible location for the ‘maternal side’ biopsy employed by Bové et al. which is a mixed tissue biopsy comprising fetal chorionic villous tissue and anchoring villi, and a layer of maternal decidual tissue. Created with Biorender.com.bMicrograph of term maternal-fetal interface demonstrating the different structure of the decidua layer (maternal) that is delivered with the placenta (fetal). Decidua contains a mix of stromal cells, leucocytes and invaded extravillous trophoblast. Tissue stained with antibodies to Cytokeratin 7, which marks placental trophoblast. Nuclei counterstained with haematoxylin. 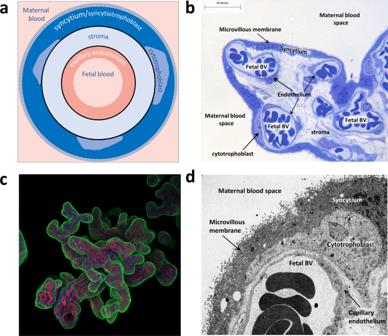Fig. 2: Cellular organisation and structure of the human placenta, demonstrating the cell layers between maternal and fetal circulations. The surface of the placenta facing the maternal blood is covered by a multinucleate syncytiotrophoblast with a microvillous surface to facilitate exchange. The syncytiotrophoblast layer is formed by the fusion of the underlying cytotrophoblast cells. Beneath this lies the stroma, which contains fibroblasts and placental macrophages, and placental blood vessels lined by endothelial cells.aDiagram of a cross-section through a placental villus, showing the fetal syncytiotrophoblast in contact with maternal blood and fetal blood in the capillary endothelium.bSemi-thin section of term placenta stained with Toluidine blue. Fetal BV; fetal blood vessel.cWhole-mount term placenta stained with lectins illustrating the syncytiotrophoblast in contact with maternal blood in green, stroma in blue and the fetal capillaries in magenta.dElectron micrograph illustrating the three main cell layers between the maternal and fetal circulations. Human subjects Where required, we have complied with all relevant ethical regulations, and informed consent was obtained from participants. Ethical approval was provided by the Northern X Regional Ethics Committee (New Zealand; NTX/12/06/057/AM09) or Southampton and Southwest Hampshire Local Research Ethics Committee (UK; 11/SC/0529). Immunohistochemistry Paraformaldehyde-fixed term human placenta-decidua biopsies were snap frozen in OCT compound, cut and subjected to heat induced antigen retrieval. Sections were blocked in 10% Normal Goat Serum and stained with 2 μg/mL cytokeratin 7 antibody (clone OV-TL 12/30, Dako Laboratories #M7018). Secondary and tertiary steps were undertaken using a Histostain-plus kit (Thermofisher Scientific). Colour was developed with AEC, and sections counterstained in Gills II Haematoxylin, prior to mounting with Aquamount. Immunofluorescence Paraformaldehyde-fixed term human placental villi were stained with FITC-Aleuria Aurantia Lectin to visualise blood vessels, Biotin Datura Stramonium Lectin with Streptavidin 680 to visualise the trophoblast and Rhodamine-labelled Pisum sativum Agglutinin which binds the stroma (all Vector Laboratories), and imaged by confocal microscopy. Electron microscopy Villous tissue from term placenta was fixed in 2.5% glutaraldehyde in 0 1 M cacodylate buffer, post-fixed in 1% osmium tetroxide and embedded in epoxy resin. Semi-thin sections were stained with 1% toluidine blue in 1% borax for examination at the light microscopic level. Ultrathin sections from suitable areas were stained with uranyl acetate and lead citrate before examining in an AEI EM6B electron microscope. Reporting summary Further information on research design is available in the Nature Research Reporting Summary linked to this article.